Dynamics of anterior–posterior axis formation in the developing mouse embryo The development of an anterior–posterior (AP) polarity is a crucial process that in the mouse has been very difficult to analyse, because it takes place as the embryo implants within the mother. To overcome this obstacle, we have established an in-vitro culture system that allows us to follow the step-wise development of anterior visceral endoderm (AVE), critical for establishing AP polarity. Here we use this system to show that the AVE originates in the implanting blastocyst, but that additional cells subsequently acquire AVE characteristics. These 'older' and 'younger' AVE domains coalesce as the egg cylinder emerges from the blastocyst structure. Importantly, we show that AVE migration is led by cells expressing the highest levels of AVE marker, highlighting that asymmetry within the AVE domain dictates the direction of its migration. Ablation of such leading cells prevents AVE migration, suggesting that these cells are important for correct establishment of the AP axis. The first days of mouse embryo development are devoted to setting aside a group of pluripotent cells, the epiblast, from two extra-embryonic lineages: the trophectoderm and primitive endoderm. Epiblast cells will give rise to all cells of the future body while both of the extra-embryonic tissues are critical to provide support for embryo development in utero and for establishing the anterior–posterior (AP) axis. It is relatively well known how these lineages become established, as embryos can be cultured, manipulated and imaged until the blastocyst stage. However, as the blastocyst implants into the uterus, it becomes inaccessible and, therefore, it has been difficult to follow the dynamics of the events leading to AP axis formation. Following implantation, the epiblast and surrounding extra-embryonic tissues undergo a burst of proliferation and transform into the egg cylinder, an elongated cup-like structure that becomes the foundation of the future body. This transformation is a highly dynamic process associated with intensive growth and changes in the shape and topology of the tissues. As a result, the epiblast becomes positioned toward the distal part of the egg cylinder, the trophectoderm-derived extra-embryonic ectoderm (ExE) locates in the proximal part, and both of these tissues become enveloped by primitive endoderm-derived visceral endoderm (VE). Around this time, AP polarity becomes defined. By embryonic day 5.5 (E5.5), a distinct group of VE cells, the anterior visceral endoderm (AVE), have assembled at the distal tip of the egg cylinder [1] , [2] . This unique group of cells will subsequently expand and undertake unilateral movement towards the proximal region of the egg cylinder to specify the site where the head will form [1] , [3] , [4] . This movement is critical for correct positioning of the AP axis. It is well-established that AVE formation is the result of a combination of inductive signalling by the transforming growth factor-β family members, Nodal and Activin [5] , [6] , [7] , and inhibitory signals originating in ExE, particularly bone morphogenetic protein 4 [8] , [9] , [10] , [11] . However, how the AVE becomes specified and the dynamics of its formation currently remain unclear. Interestingly, several recent studies indicate that expression of AVE markers such as Lefty1 [12] , [13] and Cerl [14] , [15] is initiated at the blastocyst stage, and so, earlier than previously expected. But are these cells that show early expression of AVE markers truly AVE progenitors? If so, how do they develop to contribute to the AVE? To answer these questions directly would require the visualisation and continuous tracing of the behaviour of these early expressing cells from pre- to post-implantation stages as the AVE forms. Until now, this has not been possible, because although embryo culture throughout this stage had been reported in the past [16] , [17] , [18] , [19] the reported protocols have not been widely adopted, most likely because of the lack of quantitative comparison with in vivo development and poor efficiencies of embryo survival. Most importantly, they have never been developed for high-resolution time-lapse imaging, and consequently, dynamic observations of this crucial stage of development have never been made. To build a picture of this critical pre- to post-implantation transition, we previously carried out a series of complex experiments in which individual blastocyst cells were marked, then blastocysts were transferred into foster mothers to permit further development and subsequently recovered at successive implantation stages to analyse the clonal distribution of cells [3] , [15] , [20] . This very laborious approach proved insightful and suggested a model for how the egg cylinder might emerge from the blastocyst structure, but this complex process could only be extrapolated from a limited number of static pictures. Therefore, aiming to gain better and direct insight into how the blastocyst transforms into the egg cylinder and how the AP axis forms, we designed conditions that would allow reproducible development, and importantly, four-dimensional imaging of single cell behaviour, beyond the blastocyst stage outside the mother. Here we report the step-wise development of AVE sub-domains from individual cells of the implanting blastocyst and their subsequent coalescence to form an asymmetrical domain of AVE at the distal tip of the egg cylinder. These key stages of AVE formation have been observed in real time, using our newly validated in-vitro embryo culture technique that can be used to follow the dynamics of cellular events within the embryo at post-implantation stages. We show that such in vitro -cultured and -imaged embryos develop the correct morphology and spatio-temporal expression of epiblast, trophectoderm- and primitive endoderm-derived tissue marker genes as the blastocyst grows into the egg cylinder. We also confirm that the AVE develops in accordance with 'snap-shot' observations of embryos sampled from mothers at successive implantation stages [12] , [13] , [15] , [20] , and the pattern of expression of anterior and posterior markers indicates proper establishment of the AP axis. Finally, we show that the asymmetry in the expression of AVE marker genes dictates the direction of its anterior migration. Novel culture system to follow development beyond the blastocyst stage To follow the dynamics of AVE development, we first needed to establish a reproducible system for culturing mouse embryos in vitro , which would permit time-lapse observations of the transition from the pre-implantation blastocyst to the post-implantation egg cylinder. As a starting point, we evaluated culture methods that had been reported in the 1970s [16] , [17] , [18] but not widely adopted. We found that supplementing the media with human cord serum was the key to success and permitted the development of approximately 40% of blastocysts to the egg cylinder stage on plastic culture dishes ( Supplementary Fig. S1 ; Supplementary Table S1 ). Under these conditions, the egg cylinders that developed from blastocysts in vitro were morphologically similar to egg cylinders collected from mothers, and showed the same spatial patterns of expression of the respective ExE, VE and epiblast marker genes, Cdx2, Gata4 and Oct4 ( Supplementary Fig. S1 ). However, this culture system was not suitable for our purpose, as the plastic dishes used as a platform for the embryo development were not amenable to live-imaging at cellular resolution. Moreover, we found that none of the commercially available, optically friendly culture dishes permitted correct development ( Supplementary Table S1 ). Therefore, we assessed the use of polyacrylamide hydrogels bonded to glass and overlaid with various protein coatings, as similar approaches have been successful in other cell culture systems [21] ( Supplementary Tables S1 and S2 ). We found that two variables were of particular importance for successful culture of embryos. First, the surface stiffness of the polyacrylamide hydrogel, which we optimised by varying N ′ N ′-methylenebisacrylamide and acrylamide ratios; second, its protein coating. A coating of type I rat-tail collagen allowed 87% (13/15) of embryos to attach to the matrix and 38% (5/13) to develop into egg cylinders ( Supplementary Table S2 ). In contrast, laminin or fibronectin alone were unsuitable surface coatings, but would allow 80% (12/15) of embryos to attach and 41% (5/12) to form egg cylinders when used in combination with collagen. We set out to use these collagen-coated polyacrylamide matrices to follow the cellular dynamics of an egg cylinder emergence by spinning-disc, confocal time-lapse microscopy. Typically, when zona-free E3.5 blastocysts were seeded onto the culture gels, embryos developed over 5 days following the indicated time course ( Fig. 1a–d ; Supplementary Movies 1–3 ). We confirmed the normal morphology of the egg cylinders that had developed from the blastocysts in vitro by recovering them from the gel after time-lapse imaging and staining them with the vital lipophilic dye FM4-64 to reveal individual cells by optical sectioning ( Fig. 1e ). 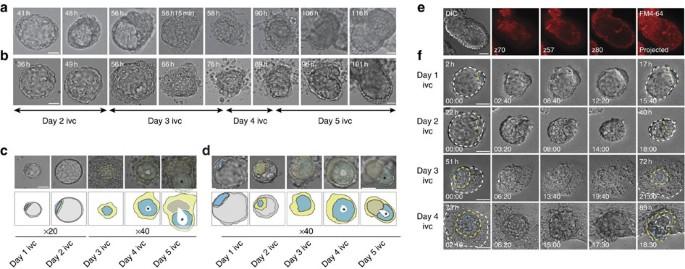Figure 1:In vitroculture of blastocysts on collagen-coated polyacrylamide matrices allows successful development to the egg cylinder stage. (a,b) DIC time-lapse observations ofin vitrodevelopment of two representative blastocysts on collagen-coated polyacrylamide gels covalently bound to a glass-bottomed dish. Each panel shows a single embryo continuously observed from the second day ofin vitroculture (ivc), until the fifth day. Panels (a) and (b) show selected frames fromSupplementary Movies 1 and 2, respectively. Elapsed developmental time from the point at which the blastocyst was placed on the gel is shown at the top of each frame. Scale bars represent 50 μm. (c,d) Development of two further representative embryosin vitroand observed using a ×40 objective. DIC images are shown alongside schematics showing different tissues: epiblast, blue; primitive/visceral endoderm, yellow; trophectoderm/ExE, grey; the pro-amniotic cavity is highlighted by an asterisk. The overlying trophectoderm is omitted from the schematics of the third and fourth day ofin vitroculture, for clarity. Development of the embryo shown in (c) is presented inSupplementary Movie 3. (e) On day 5 ofin vitroculture, the embryo shown in (d) was removed from the gel and stained with the lipophilic dye FM4-64. DIC, selected confocal stacks and projected images are shown. (f) DIC time-lapse observations during 4 days of developmentin vitro.A representative embryo is shown for each day of culture. Elapsed developmental time from the point at which the blastocyst was placed on the gel is shown at the top of the first and the last frame presented for each day. Time points at the bottom of each still represent individual time frames from time-lapse observations on the indicated day. Embryonic and extra-embryonic structures are indicated as follows: primitive endoderm (blastocyst) and visceral endoderm (egg cylinder), yellow-dashed line; trophectoderm (blastocyst) and ExE (egg cylinder), white-dashed line; epiblast, blue-dashed line. Scale bars represent 50 μm. Figure 1: In vitro culture of blastocysts on collagen-coated polyacrylamide matrices allows successful development to the egg cylinder stage. ( a , b ) DIC time-lapse observations of in vitro development of two representative blastocysts on collagen-coated polyacrylamide gels covalently bound to a glass-bottomed dish. Each panel shows a single embryo continuously observed from the second day of in vitro culture (ivc), until the fifth day. Panels ( a ) and ( b ) show selected frames from Supplementary Movies 1 and 2 , respectively. Elapsed developmental time from the point at which the blastocyst was placed on the gel is shown at the top of each frame. Scale bars represent 50 μm. ( c , d ) Development of two further representative embryos in vitro and observed using a ×40 objective. DIC images are shown alongside schematics showing different tissues: epiblast, blue; primitive/visceral endoderm, yellow; trophectoderm/ExE, grey; the pro-amniotic cavity is highlighted by an asterisk. The overlying trophectoderm is omitted from the schematics of the third and fourth day of in vitro culture, for clarity. Development of the embryo shown in ( c ) is presented in Supplementary Movie 3 . ( e ) On day 5 of in vitro culture, the embryo shown in ( d ) was removed from the gel and stained with the lipophilic dye FM4-64. DIC, selected confocal stacks and projected images are shown. ( f ) DIC time-lapse observations during 4 days of development in vitro. A representative embryo is shown for each day of culture. Elapsed developmental time from the point at which the blastocyst was placed on the gel is shown at the top of the first and the last frame presented for each day. Time points at the bottom of each still represent individual time frames from time-lapse observations on the indicated day. Embryonic and extra-embryonic structures are indicated as follows: primitive endoderm (blastocyst) and visceral endoderm (egg cylinder), yellow-dashed line; trophectoderm (blastocyst) and ExE (egg cylinder), white-dashed line; epiblast, blue-dashed line. Scale bars represent 50 μm. Full size image Dynamics of the blastocyst to egg cylinder transformation in vitro We first wished to use this new in-vitro culture/imaging system to describe the developmental events occurring as the blastocysts develop into egg cylinders ( Fig. 1f ). We observed that during the first day of in vitro culture, the blastocysts underwent expansion and contraction before thickening of the mural trophectoderm became evident during the second day. Higher resolution imaging allowed us to discern the basal lamina, separating the epiblast from the primitive endoderm at this stage (optical sections in Fig. 2a ). By the third day of culture, trophoblast cells had migrated across the collagen surface, resulting in spreading and flattening of the embryos, and typical blastocyst morphology was lost. The beginnings of the egg cylinder formation were marked on the fourth day by the appearance of VE and of ExE close to the site of attachment. The embryonic VE and the underlying epiblast then started to 'grow out' from the surface, whereas the extra-embryonic components remained firmly 'implanted' and spread out across the matrix (optical sections in Fig. 2b ). Mature egg cylinders were consistently found towards the end of day 4 or on day 5. At this stage, the epiblast developed the shape of a cup surrounding the pro-amniotic cavity and extending towards the extra-embryonic compartment. VE enveloped both the embryonic and extra-embryonic regions of such egg cylinders. 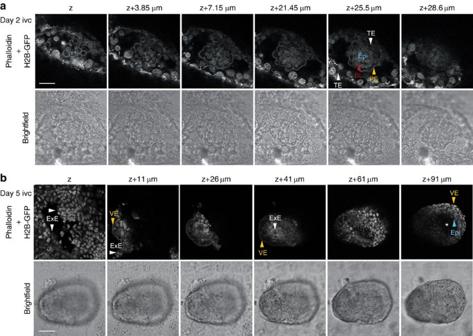Figure 2: Optical sections of embryos after 2 or 5 days ofin vitroculture. Mouse blastocysts from the H2B-GFP transgenic reporter line were cultured on polyacrylamide hydrogels coated with collagen on a 24-well glass-bottomed plate and fixed on either the second (a) or fifth (b) day ofin vitrodevelopment. Selected laser-scanning confocal z-planes are shown for each developmental stage in which both nuclei (H2B-GFP) and cortical cytoskeleton (Phalloidin) is shown merged on a grey scale. Bright-field images corresponding to each focal plane are shown beneath the fluorescent images. Scale bars shown in (a) represent 50 μm and in (b) 100 μm. Arrowheads indicate the epiblast (Epi, blue); primitive endoderm (PE, yellow); visceral endoderm (VE, yellow); trophectoderm (TE, white) and ExE (white); basal lamina (BL, red). We were unable to identify parietal endoderm or Reichert's membrane. The asterisk indicates the pro-amniotic cavity. Figure 2: Optical sections of embryos after 2 or 5 days of in vitro culture. Mouse blastocysts from the H2B-GFP transgenic reporter line were cultured on polyacrylamide hydrogels coated with collagen on a 24-well glass-bottomed plate and fixed on either the second ( a ) or fifth ( b ) day of in vitro development. Selected laser-scanning confocal z-planes are shown for each developmental stage in which both nuclei (H2B-GFP) and cortical cytoskeleton (Phalloidin) is shown merged on a grey scale. Bright-field images corresponding to each focal plane are shown beneath the fluorescent images. Scale bars shown in ( a ) represent 50 μm and in ( b ) 100 μm. Arrowheads indicate the epiblast (Epi, blue); primitive endoderm (PE, yellow); visceral endoderm (VE, yellow); trophectoderm (TE, white) and ExE (white); basal lamina (BL, red). We were unable to identify parietal endoderm or Reichert's membrane. The asterisk indicates the pro-amniotic cavity. Full size image To confirm whether the dimensions of embryos developing in vitro are similar to those developing in utero , we next used the system to culture and image the development of embryos expressing transgenes for Histone H2B-GFP [22] and Oct4ΔPE-GFP [23] (Oct4 deleted for the proximal enhancer). The former provides a marker for all nuclei, thus facilitating all cells to be followed at successive stages; the latter provides a marker to follow the pluripotent cells before the egg cylinder stage and germ cells thereafter ( Supplementary Fig. S2a,b ). We found that the embryonic and extra-embryonic compartments of the in-vitro developing egg cylinders, and the dimensions and overall shapes of the cultured embryos were comparable to embryos that had developed in utero ( Supplementary Fig. S2c,d and legend). To further assess the extent to which development in vitro resembles development in utero , we examined and compared the spatial expression of anterior and posterior markers in egg cylinders of the in vitro and in vivo cultured embryos. To this end, we cultured blastocysts derived from a transgenic reporter line in which green fluorescent protein expressed from the Cerl promoter marks the development of AVE [14] . At the fifth day of development in vitro , the expression of this AVE marker was similar to its pattern in the egg cylinders freshly collected from mothers ( Fig. 3a ). We also assessed the expression of the posterior marker, Brachyury , through in situ hybridisation and found that as in embryos developing in vivo , its transcripts were present in the opposing (posterior) side and were characteristically restricted to the embryonic/extra-embryonic boundary ( Fig. 3a ). As a further test for correct development of the anterior, we carried out co-staining for Cerl and another AVE marker, Lefty1. This revealed that these markers are co-expressed at successive stages of AVE development ( Fig. 3b,c ). Together, these results indicate that the development of AVE in vitro accords with the 'snap-shot' observations made by ourselves and by others, of embryos recovered from pregnant mothers during implantation stages [12] , [13] , [15] , [20] . Moreover, upon AVE migration, the in vitro -cultured embryos initiate the expression of Brachyury , indicating a proper establishment of AP polarity. As Brachyury expression marks the site of primitive streak formation, this suggests that embryos cultured in vitro are competent to gastrulate. 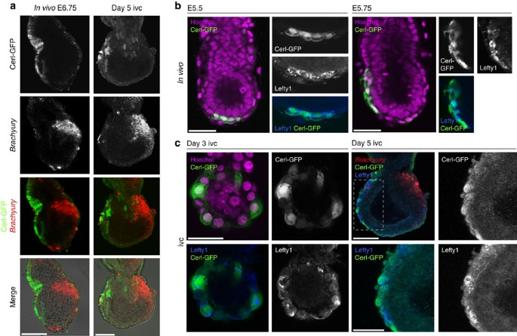Figure 3: Spatial expression of molecular markers of development ofin vitrocultured embryos. (a) Fluorescentin situhybridisation forBrachyurywith co-immunostaining for GFP in E6.5in vivo- (upper panels) and day 5in vitro-cultured (lower panels) Cerl-GFP transgenic embryos. AP patterning is faithfully recapitulated in five out of seven embryos. Scale bars represent 100 μm. (b) Co-immunostaining for Lefty1 and GFP in E5.5 and E5.75 Cerl-GFP transgenic embryos. Expression of the reporter gene is observed in the same region as another AVE-specific protein, Lefty1. Scale bars represent 50 μm. (c) Co-immunostaining for Lefty1 and GFP in day 3 and day 5in vitro-cultured Cerl-GFP transgenic embryos. The expression of Lefty1 is restricted to the GFP-positive domain throughout development. Scale bar represents 50 μm. On the fifth day ofin vitroculture (right-hand side panels),Brachyuryexpression is detected by FISH opposite to Lefty1, and Cerl-GFP domain is detected by co-immunofluorescence. Scale bars represent 100 μm. Figure 3: Spatial expression of molecular markers of development of in vitro cultured embryos. ( a ) Fluorescent in situ hybridisation for Brachyury with co-immunostaining for GFP in E6.5 in vivo - (upper panels) and day 5 in vitro -cultured (lower panels) Cerl-GFP transgenic embryos. AP patterning is faithfully recapitulated in five out of seven embryos. Scale bars represent 100 μm. ( b ) Co-immunostaining for Lefty1 and GFP in E5.5 and E5.75 Cerl-GFP transgenic embryos. Expression of the reporter gene is observed in the same region as another AVE-specific protein, Lefty1. Scale bars represent 50 μm. ( c ) Co-immunostaining for Lefty1 and GFP in day 3 and day 5 in vitro -cultured Cerl-GFP transgenic embryos. The expression of Lefty1 is restricted to the GFP-positive domain throughout development. Scale bar represents 50 μm. On the fifth day of in vitro culture (right-hand side panels), Brachyury expression is detected by FISH opposite to Lefty1, and Cerl-GFP domain is detected by co-immunofluorescence. Scale bars represent 100 μm. Full size image As a final test, we determined whether the development of exogenous, transplanted embryonic stem (ES) cells would occur correctly in embryos cultured in vitro and therefore would allow us to follow the dynamics of their contribution as the egg cylinder emerges. To this end, we aggregated ES cells expressing the marker gene, dsRed , with eight-cell stage histone H2B-GFP [24] host embryos and cultured such chimeras in vitro until the egg cylinder emerged. Our time-lapse observations revealed that the ES cells proliferated and became incorporated mostly into the epiblast rather than the VE or the ExE of the egg cylinder ( Fig. 4 ; Supplementary Movie 4 ), in accordance with their contribution in embryos developing in utero [25] . 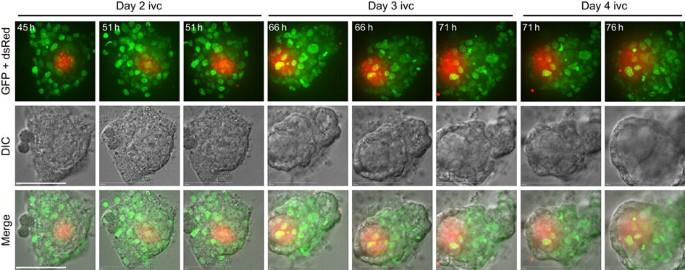Figure 4: ES cells contribute to the epiblast of chimeric embryos culturedin vitrobeyond the blastocyst stage. dsRed expression marks the ES cell line introduced into the chimera and GFP marks the host embryo. The figure displays selected frames from a time-lapse movie (Supplementary Movie 4) of a single chimera from the implanting blastocyst to the egg cylinder stage. ivc,in vitroculture. Scale bars represent 100 μm. Figure 4: ES cells contribute to the epiblast of chimeric embryos cultured in vitro beyond the blastocyst stage. dsRed expression marks the ES cell line introduced into the chimera and GFP marks the host embryo. The figure displays selected frames from a time-lapse movie ( Supplementary Movie 4 ) of a single chimera from the implanting blastocyst to the egg cylinder stage. ivc, in vitro culture. Scale bars represent 100 μm. Full size image Taken together, these results indicate that the development of embryos on collagen-coated polyacrylamide matrices permits the emergence of egg cylinders that are similar to those collected from the uteri of pregnant mothers, both in morphology and in patterns of gene expression, as well as in establishment of an AP axis as judged by the expression of both anterior and posterior markers. The proper restriction of ES cells to the epiblast when aggregation chimeras are allowed to develop in vitro is a further indication that the development in vitro recapitulates the development in utero . AVE-formation dynamics as blastocyst transforms into the egg cylinder A number of studies have attempted to relate the spatial organisation of the pre-implantation blastocyst to that of the post-implantation egg cylinder, with particular reference to the emergence of the AVE and thus of the AP axis of the embryo [13] , [14] , [15] . However, due to the necessity of transferring pre-implantation embryos to foster mothers to allow their further development, the continuity of these processes was until now impossible to determine. Thus, we next evaluated whether our new in vitro culture system in combination with time-lapse imaging could enable us to follow AVE development as the blastocysts grew into egg cylinders. We collected E3.5 blastocysts from female F1 mice mated with Cerl-GFP male mice and seeded them onto the collagen-coated polyacrylamide hydrogels. We recorded Cerl-GFP expression during continuous development in vitro from its onset in the blastocyst until its consolidation in the AVE ( Supplementary Fig. S3a ; Supplementary Movie 5 ). Detailed analyses of these movies allowed us to register the positions of Cerl-GFP-expressing cells in multiple focal planes as development progressed ( Fig. 5 ; Supplementary Movie 6 ). This revealed the onset of Cerl-GFP expression in one or two cells of the inner cell mass in the free-floating blastocyst (not shown), in accordance with previous observations [13] , [15] . We found that at this stage, the Cerl-GFP expression was transient, as when the blastocyst first attached to the culture matrix, the Cerl-GFP expression was not evident. However, Cerl-GFP expression appeared in single primitive endoderm cells and progressively increased in intensity once the blastocysts had completely flattened onto the matrix surface ( Fig. 5 , Day 3). With time, other primitive endoderm cells surrounding the epiblast began to express Cerl-GFP. These Cerl-GFP-expressing cells were found both in the vicinity of the first expressing cell and in another region within the primitive endoderm ( Fig. 5 , Day 3). Interestingly, we observed that the emergence of the egg cylinder structure from the flattened blastocyst coincided with the consolidation of the Cerl-GFP-expressing cells into the early AVE domain ( Fig. 5 , Day 3 to start of Day 4). On the fourth day of culture, as the egg cylinder grew, this Cerl-GFP cluster of cells could be seen to occupy only one side of the embryo ( Fig. 5 , Day 4). We noticed that the expression of Cerl-GFP was typically heterogeneous in intensity, with some cells showing much higher expression than others ( Fig. 5 , Supplementary Fig. S3c ). 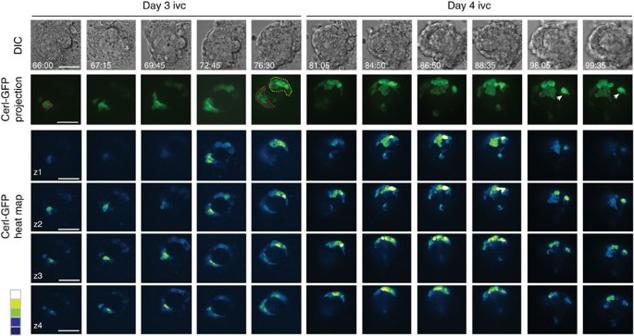Figure 5: Time-lapse-imaging of blastocysts culturedin vitroreveals the formation of the AVE. Day 3: within 6 h of the onset of expression of Cerl-GFP in a single cell (red-dotted lines, top panel), two opposing domains of Cerl-GFP-expressing cells can be observed in the primitive endoderm (red- and yellow-dotted lines;Supplementary Movie 6). Day 4: Cerl-GFP-expressing cells become progressively restricted to one side of the nascent egg cylinder. Among these, the brightest cell (white arrow) becomes progressively distant from the central domain. Scale bars represent 100 μm. The lower panels represent heatmaps of the intensity levels of Cerl-GFP on four different topical sections. The colour bar on the left-hand side of the bottom panel is the look-up table for GFP intensity in which white is the brightest. The GFP fluorescence is a maximum intensity projection over the z-axis of confocal sections. ivc,in vitroculture. Figure 5: Time-lapse-imaging of blastocysts cultured in vitro reveals the formation of the AVE. Day 3: within 6 h of the onset of expression of Cerl-GFP in a single cell (red-dotted lines, top panel), two opposing domains of Cerl-GFP-expressing cells can be observed in the primitive endoderm (red- and yellow-dotted lines; Supplementary Movie 6 ). Day 4: Cerl-GFP-expressing cells become progressively restricted to one side of the nascent egg cylinder. Among these, the brightest cell (white arrow) becomes progressively distant from the central domain. Scale bars represent 100 μm. The lower panels represent heatmaps of the intensity levels of Cerl-GFP on four different topical sections. The colour bar on the left-hand side of the bottom panel is the look-up table for GFP intensity in which white is the brightest. The GFP fluorescence is a maximum intensity projection over the z-axis of confocal sections. ivc, in vitro culture. Full size image The analyses of these time-lapse observations revealed that Cerl-GFP expression appeared in two clear separate domains in 7 out of 11 embryos studied. This resembles the pattern of Cerl-GFP expression previously reported in snapshot observations of embryos developing in utero [15] (compare Cerl-GFP expression patterns in vitro and in vivo in Supplementary Fig. S3b ). We observed that, as development progressed, these two Cerl-GFP-expressing domains always coalesced at the distal part of the egg cylinder. Either the first ('older') or the second ('younger') Cerl-GFP domain to arise could develop into the brightest part of the merged domains ( Supplementary Fig. S3c ). In all cases studied, the outcome was a cluster of cells at the distal part of the egg cylinder that showed a range of Cerl-GFP expression as judged by fluorescence levels. These results indicate that the AVE originates in the implanting blastocyst, but subsequently, an additional domain of cells acquires the AVE characteristics. These 'older' and 'younger' domains coalesce as the egg cylinder emerges from the blastocyst structure. Asymmetry of the AVE The time-lapse observations indicated that on day 4 of in vitro culture, one cell within the AVE domain at the distal tip of the egg cylinder showed higher levels of Cerl-GFP expression than its neighbours and was set apart from them ( Fig. 5 ). This prompted us to examine if this heterogeneity of Cerl-GFP levels also exists in vivo and, if so, whether it is of physiological relevance to the subsequent migration of the AVE. We collected embryos that already had AVE positioned at the distal tip of the egg cylinder, and first examined the Cerl-GFP expression levels. We observed a domain of three to nine cells clearly expressing Cerl-GFP at the distal tip of the embryo and positioned slightly, but clearly, towards one side before AVE movement commenced ( Fig. 6a , n =6), in agreement with previous observations [9] , [14] . We found that a cell expressing higher levels of Cerl-GFP was positioned ahead of other Cerl-GFP-positive cells ( Fig. 6a,b ; five out of six embryos), suggesting it could be leading migration of the AVE domain. We also observed that this most anteriorly located Cerl-GFP-expressing cell extended projections towards the anterior region and initiated migration in that direction ( Fig. 6a , arrows, Supplementary Movie 7 ). To verify this observation, we analysed the dimensions of these cells by measuring their maximum length and width in relation to their long axis in in-vitro -developed egg cylinders and freshly collected embryos. This revealed that the most anteriorly located Cerl-GFP-expressing cell became significantly more elongated with time in comparison with the cuboidal cells following its migratory trajectory, and that this was the case for both embryos developing in vivo or in vitro ( Fig. 6c–e ). Quantification of Cerl-GFP fluorescence indicated that the greater the intensity, the more elongated the cell ( Fig. 6e ). These results indicate an asymmetry in the expression of the AVE marker gene and suggest that the cell expressing Cerl-GFP at the highest levels might be the cell that leads AVE migration. 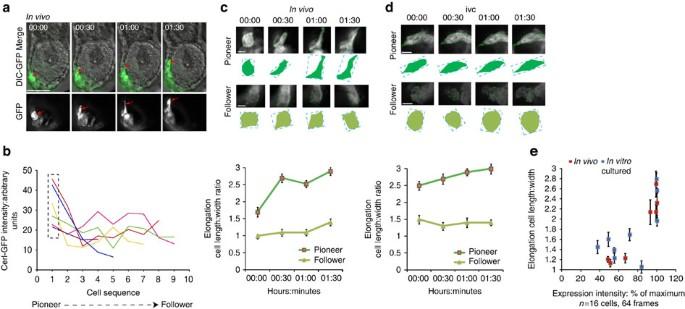Figure 6: The most anterior cell expressing the highest levels of Cerl-GFP leads migration of the Cerl-GFP-expressing cells in a collective domain. (a) The putative leading AVE cell (red arrow) in an E5.5 embryo extends protrusions towards the prospective anterior region and migrates over the 2 h of imaging shown (Supplementary Movie 7). (b) Fluorescence intensity levels (arbitrary units) of Cerl-GFP-expressing cells in six E5.5 embryos. The leading AVE cell (number 1) is always amongst the strongest Cerl-GFP-expressing cells. Cerl-GFP-expressing cell shape was monitored over the course of 2 h of live imaging in freshly collected 'in vivo' embryos (c) andin vitro-cultured embryos. Scale bars represent 20 μm. (d) In each case—examples of strong Cerl-GFP-expressing leading AVE cells and weaker-expressing followers are shown. Following repeated tracings of cell shape, rectangles of best fit were constructed around the cell boundaries for all four time points over the 2-h period. (e) Each set of rectangles represents the changing cell shape over time—the average length to width ratio was calculated and plotted against the average intensity of Cerl-GFP expression for each cell. A total of 16 cells were analysed over 64 time points. Figure 6: The most anterior cell expressing the highest levels of Cerl-GFP leads migration of the Cerl-GFP-expressing cells in a collective domain. ( a ) The putative leading AVE cell (red arrow) in an E5.5 embryo extends protrusions towards the prospective anterior region and migrates over the 2 h of imaging shown ( Supplementary Movie 7 ). ( b ) Fluorescence intensity levels (arbitrary units) of Cerl-GFP-expressing cells in six E5.5 embryos. The leading AVE cell (number 1) is always amongst the strongest Cerl-GFP-expressing cells. Cerl-GFP-expressing cell shape was monitored over the course of 2 h of live imaging in freshly collected ' in vivo ' embryos ( c ) and in vitro -cultured embryos. Scale bars represent 20 μm. ( d ) In each case—examples of strong Cerl-GFP-expressing leading AVE cells and weaker-expressing followers are shown. Following repeated tracings of cell shape, rectangles of best fit were constructed around the cell boundaries for all four time points over the 2-h period. ( e ) Each set of rectangles represents the changing cell shape over time—the average length to width ratio was calculated and plotted against the average intensity of Cerl-GFP expression for each cell. A total of 16 cells were analysed over 64 time points. Full size image AVE asymmetry dictates the direction of its migration We wished to determine whether the asymmetric distribution of cells strongly expressing Cerl-GFP is important for the subsequent directionality of AVE migration. To this end, we laser ablated individual cells within the AVE domain showing differences in the levels of Cerl-GFP expression and followed the consequences for AVE behaviour. Having ensured that laser ablation of a target cell had no effects upon neighbouring cells ( Supplementary Fig. S4a,b ), we first ablated the leading AVE cell, which showed the highest level of Cerl-GFP expression ( Fig. 7 ). This had a dramatic effect on AVE behaviour. In all 14 embryos examined, ablation of this leading cell abolished the migration of all AVE cells and prevented expansion of the AVE domain ( Fig. 7a ; Supplementary Movies 7 and 8 ; Supplementary Fig. S4c ). 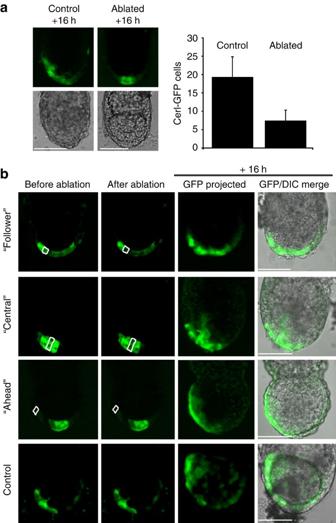Figure 7: AVE migration requires leading AVE cells. (a) Projected confocal images of control embryos (left panels) and an embryo in which the leading AVE cell was ablated by laser-irradiation (right panels,Supplementary Movie 8) 16 h after ablation. Migration of the Cerl-GFP expressing cells is prevented when the leading AVE cell is ablated. Numbers of Cerl-GFP expressing cells in control and leading cell-ablated embryos were quantified 16 h after ablation: Ablation of leading cells prevents expansion of the Cerl-GFP-expressing domain. (b) Consequences of cell ablation for AVE migration and expansion: cell ablation immediately behind the leading cell, in the central section of the AVE, and in a region of visceral endoderm anterior to the AVE. Images of Cerl-GFP expression are taken immediately before and after ablation, and 16 h later. Scale bars represent 100 μm. To determine to what extent the failure of AVE migration reflected some unique quality of its leading cell or a general property of the entire AVE domain, we next ablated individual cells at different positions in the AVE. We found that ablation of the cell immediately following the pioneer was also effective in preventing AVE migration; however, it still allowed an increase in the number of the Cerl-GFP cells ( Fig 7b ; n =10; Supplementary Fig. S4d ). In contrast, ablation of a cell in the central domain of the trailing group of Cerl-GFP-expressing cells permitted anterior migration and AVE expansion, although to a slightly lesser extent than in control embryos ( Fig. 7b ; n =5; Supplementary Fig. S4e ). Ablation of Cerl-GFP-negative cells in the VE ahead of the leading cell had no effect on either AVE migration or its expansion, suggesting that cell ablation per se is not likely to provide a physical barrier to cell migration ( Fig. 7b , n =5). These results indicate that AVE migration is led by cells expressing the highest levels of AVE marker genes and therefore, suggest that the asymmetry within the AVE domain drives the direction of its migration. The fact that ablation of a single leading cell or its immediate follower could prevent AVE migration suggests that AVE migrates as a continuous sheet of cells, and that this is important for the correct establishment of the AP axis. Figure 7: AVE migration requires leading AVE cells. ( a ) Projected confocal images of control embryos (left panels) and an embryo in which the leading AVE cell was ablated by laser-irradiation (right panels, Supplementary Movie 8 ) 16 h after ablation. Migration of the Cerl-GFP expressing cells is prevented when the leading AVE cell is ablated. Numbers of Cerl-GFP expressing cells in control and leading cell-ablated embryos were quantified 16 h after ablation: Ablation of leading cells prevents expansion of the Cerl-GFP-expressing domain. ( b ) Consequences of cell ablation for AVE migration and expansion: cell ablation immediately behind the leading cell, in the central section of the AVE, and in a region of visceral endoderm anterior to the AVE. Images of Cerl-GFP expression are taken immediately before and after ablation, and 16 h later. Scale bars represent 100 μm. Full size image Studies of the genesis of AP polarity in the mouse embryo have been restricted by the inaccessibility of the embryo during the pre- to post-implantation transition when this primary body axis becomes established. To overcome this difficulty, we have developed an in-vitro culture system that is compatible with time-lapse confocal microscopy to directly visualise how the AP axis emerges as the egg cylinder grows out of the blastocyst structure. Several lines of evidence indicate that this new approach for in vitro culture and imaging recapitulates development outside the body of the mother. First, embryos developing in vitro acquire the correct morphology and spatio-temporal expression patterns of key marker genes, indicating proper organisation of the epiblast, trophectoderm- and primitive endoderm-derived tissues in the egg cylinder. Second, they undergo rapid growth, concomitant with the formation of the proamniotic cavity, as is the case in embryos developing in the mother. Third, they develop the AVE in accordance with snapshot observations of embryos sampled from mothers at successive implantation stages [13] , [15] , [20] . Fourth, upon AVE migration, they initiate expression of the posterior marker, Brachyury , indicating proper establishment of AP polarity and competence to initiate gastrulation. Fifth, exogenous ES cells become incorporated into the appropriate tissues of the egg cylinder as it develops in vitro. Together, these results indicate that this new in-vitro culture/imaging system provides a reliable in vitro platform that recapitulates development in the uterus and enables us to follow the step-wise development of AP polarity in relation to egg cylinder morphogenesis. The future use of this platform should allow further characterisation of the cellular interactions between different lineages as the blastocyst transforms into the egg cylinder. The ability to culture mouse embryos on collagen-coated polyacrylamide matrices enabled us to follow the dynamics of AVE formation by time-lapse confocal microscopy. We show that the first cells to express Cerl-GFP develop in the inner cell mass of the pre-implantation blastocyst, but that this expression is only transient. Cerl expression becomes again evident in the primitive endoderm as the blastocyst 'implants', that is, after the trophectoderm cells have spread out on the culture substrate and the blastocyst is flattened. We show that this early expression continues, but also additional cells start to express the AVE markers. Typically, these two, 'older' and 'younger' AVE domains become consolidated by the time the egg cylinder emerges. These findings are in agreement with, and provide an explanation to, our previous snap-shot observations [15] and also support a recent report indicating that cells which start to express another AVE marker, Lefty1, in the implanting blastocyst participate in establishing the AVE [13] . As confirmation of this, our analyses of fixed embryos that develop either in vivo or in vitro indicate that the expression domains of Cerl and Lefty1 are coincident and lie opposite the posterior expression domain of Brachyury . It is important to note that, although we show that Cerl-GFP expression is initiated in individual blastocyst cells, it remains unknown whether these cells arise stochastically or in relation to some feature of the blastocyst's development, an interesting topic for future detailed investigation. Once the AVE domains have consolidated at the distal tip of the egg cylinder, we find that cells that express the AVE markers at higher levels than their neighbours lead the AVE migration process. This result is in agreement with recent findings that AVE cells are migrating actively rather than being pushed by other VE cells [26] , [27] . This is also in accord with studies showing that embryos carrying mutations in genes essential for cell migration exhibit a defective AVE movement [28] . Our results indicate that the integrity of cells that lead AVE migration and their surrounding community is required for the migratory process. This is because ablation of both the leading and following cells prevents AVE migration and expansion. In other words, our results suggest that AVE migration is a collective process and requires the group of AVE cells to act as a migratory community. However, we show that ablation of a central cell within the AVE domain and expressing its markers less intensively still permits considerable AVE migration and expansion. Taken together, these results point to two broad classes of cells within the AVE, one group that leads to the migration and another that might be carried along by this process. These findings echo a recent report, which showed that following genetic ablation of Lefty1-expressing cells soon after embryo implantation, the AVE was formed but failed to migrate [13] . Therefore, these two studies that analyse the expression of different AVE markers in embryos cultured either in vitro or in utero each suggest that the anterior migration of the AVE is guided by an independent sub-set of AVE cells. Although Cerl-GFP expression is an excellent marker of the AVE, Cerl expression on its own is not essential for the development of the AP axis [29] , which requires both Cerl and Lefty1 acting together [30] . At present, we cannot determine unequivocally whether the differing cellular behaviour we assign to AVE cells is a specific consequence of differential levels of Cerl expression or rather a more general property of cells marked in this way. Several possibilities could account for why the highest Cerl-expressing cells might act as pioneers in AVE migration. It might be that, within the AVE domain, these are the cells that are the most responsive to an attractant or cue. In such a case, the leading AVE cells would be passive responders to external signals rather than having their pioneer properties determined by the high level of Cerl expression. Moreover, it is possible that the asymmetry within the AVE would result in its unidirectional migration in response to a symmetric signal originating, for example, from the ExE [8] , [9] , [10] , [31] , [32] . Alternatively, by expressing the highest levels of Cerl and Lefty1, which are Nodal antagonists, the leading AVE cells and their immediate neighbours would suppress Nodal activity in their vicinity, thus facilitating a stepwise migration. Any asymmetry in the levels of Cerl expression could be reinforced by such a process and migration would proceed unidirectionally. Understanding whether these or other mechanisms drive AVE migration will require gaining greater understanding of the cell biology of these processes. The accessibilty of embryos at this stage of development for experimentation opens up real possibilities for achieving such goals. Embryo collection, culture and staining F1 (C57BL/6XCBA) blastocysts from either wild-type or appropriate transgenic matings (as indicated in the text) were collected into M2 medium with 4 mg ml −1 of bovine serum albumin as described previously [15] , [20] . Zona pellucidae were removed by treatment with acidic Tyrode's solution as described previously [15] . After recovery, embryos were were seeded in single wells of 24-well plates in 400 μl of in-vitro culture medium 1 (IVC1: CMRL-1066 (Invitrogen) supplemented with 200 mM L-glutamine (Invitrogen), 100 mM sodium pyruvate (Invitrogen), penicillin and streptomycin (Invitrogen), and 20% fetal calf serum (FCS, Invitrogen) either in plastic tissue culture dishes or on polyacrylamide matrices (see below). For plastic tissue culture dishes, drops of 5 μl were used. On the evening of day 2, the medium was replaced by mouth pipetting with in-vitro culture medium 2 (IVC2), which is identical to IVC1, except for the serum component for which we used 20% human cord serum (HCS, Addenbrokes Hospital, Cambridge, UK). IVC2 media was replaced on a daily basis for the remainder of the culture. For post-implantation studies, E5.5 embryos were collected from F1 females mated with Cer-l-GFP males and cultured in IVC2. All embryo cultures were performed at 37 °C in a 5% CO 2 atmosphere. The fluorescent in-situ hybridisation was performed as described before [33] . Immunostaining was carried out as previously described [15] . Polyacrylamide gels for embryo culture Polyacrylamide gels of characterised surface stiffness, covalently bonded to glass substrates, have been used to allow the mouse embryo culture in well plates and petridishes, and simultaneous time-lapse confocal imaging. Circular grade 1 borosilicate glass coverslips (Menzel-Gläser, Thermo Scientific) were cleaned in a 0.1-M sodium hydroxide solution (>98%, Sigma-Aldrich). Successive dip-coating in APTMS (97%, Sigma-Aldrich) and 0.5% glutaraldehyde solutions ( ∼ 50% solution, Fluka/Biochemika, Sigma-Aldrich) were then carried out, with wash-steps in distilled water after each APTMS and glutaraldehyde treatment. Polyacrylamide gel solutions were made containing varying concentrations of N , N '-methylenebisacrylamide solution (2% in water, Fluka/Biochemika, Sigma-Aldrich), from 0.02 to 0.5%, and 10% acrylamide solution (40% in water), Fluka/Biochemika, Sigma-Aldrich. Polyacrylamide gel was polymerised using 10% ammonium persulphate solution (98%, Sigma-Aldrich) in distilled water (1:167 volume), and NNN '-M-Tetramethylethyldiamine (TEMED; Sigma-Aldrich; 1:250 volume). Initial screening of embryo attachment was carried out using gels varying in N ′ N ′-methylenebisacrylamide concentration, but data reported is from embryos cultured on hydrogels of 0.3% N ′ N ′-methylenebisacrylamide concentration. Polyacrylamide surfaces were coated with the extracellular matrix component, collagen. A 0.2 mg ml −1 water solution of type I rat-tail collagen (9.92 mg ml −1 , BD Bioscience) was attached to the polyacrylamide gels using a 0.5 mg ml −1 in water solution of ultraviolet light-activated heterobifunctional molecule, sulfo-SANPAH (Pierce Biotechnology). The stainless steel mould for moulding gels into the correct shape was a proprietary design and manufactured by the Precision Manufacturing Centre (University of Nottingham). The mould was fabricated from 6-mm thick stainless steel. Embryos were cultured in one large cylindrical well in the centre of the gel (1130 μm diameter, 300 μm height). All wells have a base thickness from 100 μm up to 500 μm. To increase the imaging resolution at ×40 magnification, 24-well glass bottom well plates were used (PAA Laboratories GmbH, Austria). These imaging plates were already pre-functionalised with amino groups. Functionalising the imaging surface of the wells with polyacrylamide gels was carried out by applying 100 μl of 0.5% glutaraldehyde solution, then washing with distilled water. A volume of 10 μl of polyacrylamide gel solution was then applied to the imaging surface in the well. A grade 1 circular glass coverslip of 12-mm diameter (Menzel-Gläser, Thermo Scientific) was then placed on top of the gel solution. Once the gel had cured, the coverslip was removed. The method of functionalisation of the polyacrylamide gels in well plates with type I rat-tail collagen is the same as for individual gels. Time-lapse confocal imaging Time-lapse imaging during in vitro culture and following laser ablation of selected cells (see below) was performed using a confocal spinning-disc microscopy system (Intelligent Imaging Solutions). Confocal images were acquired with a QuantEM:512SC camera (Photometrics) and wide-field images on the same microscope with a CoolSnapHQ camera (Photometrics). Objectives used were a ×20 Air EC Plan Neofluar, NA 0.5, and a ×40 Air EC Plan Neofluar, NA 0.75 (Zeiss). Image stacks with 3.5 or 5 μm z-planes were captured every 12–30 min, scanning up to 100 μm up to the pre-egg cylinder stage, and up to 150 μm in the egg cylinder stage. Imaging had to be interrupted for changing medium and adjusting to the best focal plane and therefore, the data provided from time-lapse observations are often a compilation of several captures. Image processing and analysis was performed with Slidebook 5.0.0.20 or superior Image J and Adobe Photoshop. Laser ablation Elimination of the selected cell by laser irradiation was performed with an Olympus inverted FV1000 microscope with the 405-nm laser irradiating for 500 ms in the selected area. Confocal images of embryos were captured before and after ablation, and following 16 h of culture using the same system. Where indicated, fluorescence intensity was measured using ImageJ software. Animals Animals were maintained in the Animal Facility of Gurdon Institute at 12:12 light cycle and provided with food and water ad libitum . All experiments were conducted in compliance with Home Office regulations. How to cite this article: Morris, S. A. et al . Dynamics of anterior–posterior axis formation in the developing mouse embryo. Nat. Commun. 3:673 doi: 10.1038/ncomms1671 (2012).